Observation of soliton compression in silicon photonic crystals Solitons are nonlinear waves present in diverse physical systems including plasmas, water surfaces and optics. In silicon, the presence of two photon absorption and accompanying free carriers strongly perturb the canonical dynamics of optical solitons. Here we report the first experimental demonstration of soliton-effect pulse compression of picosecond pulses in silicon, despite two photon absorption and free carriers. Here we achieve compression of 3.7 ps pulses to 1.6 ps with <10 pJ energy. We demonstrate a ~1-ps free-carrier-induced pulse acceleration and show that picosecond input pulses are critical to these observations. These experiments are enabled by a dispersion-engineered slow-light photonic crystal waveguide and an ultra-sensitive frequency-resolved electrical gating technique to detect the ultralow energies in the nanostructured device. Strong agreement with a nonlinear Schrödinger model confirms the measurements. These results further our understanding of nonlinear waves in silicon and open the way to soliton-based functionalities in complementary metal-oxide-semiconductor-compatible platforms. Major breakthroughs in metrology [1] , ultrafast optics [2] , medical physics [3] and optical communications [4] that occurred over the past decades were the direct result of a deeper understanding of nonlinear optical waves in guided media. The most common media in these experiments are optical fibres or photonic crystal fibres made of silica glass. These materials, however, are not suitable for photonic integration and the search for alternative platforms, such as plasmonics [5] , high index glasses [6] and semiconductors [7] , has inspired intense research in recent years. The silicon semiconductor is of special interest due to the potential of monolithically integrating micro-electronics and photonics in a chip-scale complementary metal-oxide-semiconductor (CMOS) platform [8] . Moreover, due to the subwavelength confinement of light in the high-index semiconductor material, the energy required for these nonlinearities can reach sub-picojoule thresholds [9] , [10] , [11] . With the demonstration of hybrid opto-electronic chips in a silicon commercial foundry only last year [12] , our understanding of nonlinear wave dynamics in nanostructured silicon waveguides is critical to the continued development of dense photonic integration. One of the most fundamental nonlinear processes in optical systems is the soliton, which has already demonstrated key breakthrough applications such as supercontinuum generation [13] , imaging [14] and optical pulse compression in fibres [15] , [16] . Solitons are self-reinforcing localized waves that occur in a wide variety of nonlinear physical systems, including ion plasmas, neural networks [17] , water surfaces [18] , optical fibres [15] and cavities [19] . In the optical domain, solitons exhibit invariant or recurrent propagation behaviour resulting from the precise interaction of linear group velocity dispersion (GVD) and nonlinear self-phase modulation (SPM) [20] , [21] . Periodic dielectric media are a particularly attractive platform to observe solitons on a chip scale [22] , [23] as they can be designed for very high, very low, positive and negative dispersion values [24] (for example, up to five orders of magnitude higher than in fibre). This fact, combined with the possibility of enhancing the nonlinear effects by using slow light [25] , [26] , facilitates soliton evolution on sub-millimetre length scales. A characteristic signature of solitons is the temporal compression of the optical pulse due to the formation of higher-order solitons. Alternative non-soliton compression schemes separating out the nonlinear and linear elements have also been demonstrated [27] , [28] . Higher-order soliton pulse compressors have been demonstrated in glass fibre [15] , periodic fibre Bragg gratings [29] , [30] and on-chip in two-photon absorption (TPA)-free semiconductors [10] , [22] , [23] . While solitons in glass can couple electromagnetic energy to Raman vibrations [31] , semiconductors exhibit completely different higher-order nonlinearities, including multiphoton absorption and free carriers. These latter nonlinear effects can give rise to pulse asymmetry and acceleration, only identified in semiconductors this year [10] , [23] , [32] . Although it has been theoretically predicted that picosecond higher-order soliton compression is also possible in silicon [33] , [34] , there have been no such demonstrations to date. In order to understand the behaviour of solitons in silicon, it is critical to acknowledge that TPA and free-carrier effects play very different roles in the dynamics, even though they are linked. The first impact of TPA is to reduce the desirable SPM nonlinearity, requiring more power to counterbalance dispersion. Ultimately, the TPA caps the peak power in the system, essentially removing a critical parameter to control the soliton dynamics. More importantly, the free carriers generated by the TPA process perturb the optical soliton, and induce a blue shift, thus greatly modifying the canonical soliton evolution described by the simple picture of Kerr and GVD. Soliton-like propagation of femtosecond pulses in silicon channel waveguides has been observed through spectral measurements [35] and cross-correlation [36] . From a physics perspective, in the femtosecond regime of the latter work, no acceleration was observed as longer (picosecond) pulses are required for the non-instantaneous response of the free carriers to accumulate. The extremely large dispersion of periodic media [25] , three orders of magnitude larger than channel waveguides [36] , uniquely enables solitons with picosecond pulses, and they are consequently a favourable platform to demonstrate accelerating solitons. From a technological perspective, while there has been significant progress in on-chip femtosecond sources [37] , many nonlinear experiments rely on femtosecond pulses from bulk Ti:Saph lasers [1] , [2] , [35] that are incompatible with photonic integration. The recent demonstration of a compact laser in silicon photonic crystals offers the exciting possibility of integrating an on-chip light source in silicon [11] . Here by making use of a 396-μm-long dispersion-engineered slow-light photonic crystal waveguide (PhC-wg), we have overcome the challenges of TPA and free carriers to observe soliton compression of picosecond pulses in silicon. In order to measure the sub-pJ soliton dynamics, we have constructed an ultra-sensitive frequency-resolved electrical gating (FREG) [38] apparatus, providing us with a simultaneous measurement of the spectral and temporal domains of the optical pulses in the nanophotonic waveguides. In addition to spectral and temporal information, our measurements provide phase information on the pulses, which is crucial to explaining the free-carrier-induced temporal features. The experimental results are in very good agreement with nonlinear Schrödinger modelling. We directly measure the acceleration of pulses and confirm by simulation that this acceleration is greater than that in equivalent TPA-free media due to significantly stronger free-carrier effects in our silicon system. These results provide the key insights into nonlinear wave propagation in a CMOS-compatible platform, opening the route to soliton-based functionality in integrated photonic chips. Nonlinear wave propagation in glass and semiconductors The illustrations in Fig. 1a,b provide an insight into the semiconductor soliton regime presented in this paper relative to previous observations in glass media [15] , [29] , [39] . In the canonical case, when only SPM and GVD are present, higher-order solitons are expected to exhibit periodic evolution along the propagation direction, and experience temporal compression at an early stage along the soliton period [40] , [41] , [42] . At the point of maximum compression, shown as the narrow green pulse at the waveguide output in Fig.1a , the higher-order soliton is expected to exhibit higher intensity than the input pulse, with the same amount of energy contained in a shorter pulse. Nevertheless, aside from SPM and GVD, both in glass media and in semiconductors, higher-order effects, which can include multiphoton absorption, free carriers, or Raman, among others, alter the soliton evolution. 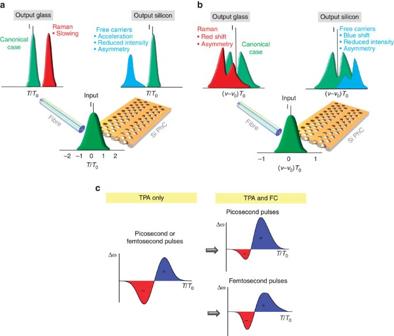Figure 1: Schematic illustrating the differences between different soliton regimes. (a) Time domain behaviour of higher-order soliton compression in glass (Raman) and silicon (free carriers) with anomalous dispersion. (b) Representation of the spectral domain with red Raman (glass) and blue free-carrier shifts (silicon) of the pulse energy. (c) The nonlinear chirp with TPA only (left panel) roughly corresponds to the canonical case. In the presence of free carriers, picosecond pulses accumulate significant blue shift. In contrast, the chirp of femtosecond pulses is relatively unaffected due to their short duration. As a consequence, picosecond pulses exhibit greater acceleration. Figure 1: Schematic illustrating the differences between different soliton regimes. ( a ) Time domain behaviour of higher-order soliton compression in glass (Raman) and silicon (free carriers) with anomalous dispersion. ( b ) Representation of the spectral domain with red Raman (glass) and blue free-carrier shifts (silicon) of the pulse energy. ( c ) The nonlinear chirp with TPA only (left panel) roughly corresponds to the canonical case. In the presence of free carriers, picosecond pulses accumulate significant blue shift. In contrast, the chirp of femtosecond pulses is relatively unaffected due to their short duration. As a consequence, picosecond pulses exhibit greater acceleration. Full size image In glass media, intrapulse Raman scattering plays the most important role among the higher-order effects [39] , [40] . For ultrashort femtosecond pulses, the blue components of the pulse provide gain to the red components ( Fig. 1b ). As a consequence, the pulse red shifts, and for the short propagation lengths considered here, the amplitude of the soliton does not change. For longer lengths, the soliton will decay due to energy dissipation through Raman effects or linear loss [31] . As bright solitons occur in media with anomalous dispersion, where low-frequency (red) components travel slower than high-frequency (blue) components, the Raman-induced red shift results in the pulse travelling more slowly ( Fig. 1a ). The observations of soliton compression presented in this paper unveil a significantly different soliton regime. In the canonical case, the behaviour would be similar to that in glass media, only that the enormous GVD achievable in photonic crystal waveguides and the larger Kerr parameter of silicon would enable the compression to occur at reduced length scales. In practice, however, the presence of TPA and free carriers in silicon drastically change the picture. Figure 1a shows a schematic of the temporal behaviour in the silicon PhC-wg. The output pulse exhibits asymmetry due to free-carrier dispersion (FCD) and absorption (FCA) and an intensity decrease due to TPA. Owing to free-carrier frequency blue shift from the FCD, the pulse undergoes acceleration in the anomalous medium and arrives before the canonical soliton in time. Figure 1b shows the corresponding properties in the frequency domain. Note that free carriers are also generated in TPA-free semiconductors via a three-photon absorption (3PA)-induced process. However, the free-carrier density observed in our silicon experiment ( N c ~10 17 cm −3 ) exceeds that observed in the TPA-free experiments [10] , [22] by an order of magnitude at similar intensities, leading to much stronger interaction between the optical pulse and the free carriers in silicon. This is shown directly by the large acceleration observed in our experiments. An important point not yet discussed in the literature is the critical role played by photonic crystals in observing free-carrier-induced acceleration. Whereas Raman processes typically require pulses in the femtosecond range for efficient intrapulse scattering [31] , in contrast, free-carrier effects require longer pulses in time. Physically, this is explained by considering that the energy in the pulse tail needs to experience the free carriers generated by the leading edge in order to undergo a blue shift. Figure 1c illustrates the nonlinear chirp corresponding to picosecond (top) and femtosecond (bottom) pulses in silicon (see Methods). The picosecond pulses clearly blue-shift significant portions of their energy, whereas the femtosecond pulses more closely resemble the TPA only case. Soliton dynamics in silicon The propagation of picosecond pulses through a silicon waveguide can be modelled with the following nonlinear Schrödinger equation (NLSE) modified to include free-carrier effects: where A(z,t) is the slowly varying amplitude of the pulse, with P 0 being the pulse peak power P 0 = |A| 2 , α l represents the linear loss, β i the i th -order dispersion, γ eff and α TPA,eff are, respectively, the effective nonlinear SPM parameter and the effective TPA parameter, k c,eff is the FCD and σ eff is the FCA. Here we are using a slow-light PhC-wg and, as a consequence of the intensity enhancement generated by slow light, all the effects in this equation scale with the slow-down factor S=n g /n 0 . While the slow-light physically enhances the intensity of the field, we adopt a notation where this scaling is included in the coefficients. The effective nonlinear and TPA parameters scale as γ eff =γ S 2 =( n 2 k 0 /A eff ) S 2 , and α TPA,eff =( α TPA,bulk /A eff ) S 2 , respectively, with the bulk coefficients n 2 =6 × 10 −18 m 2 W −1 and α TPA,bulk =8 × 10 −12 m W −1 (ref. 43 ). The k c,eff and σ eff parameters scale with S : σ eff = σS =1.45 × 10 −21 S m 2 and k c,eff = k c S=−4.5 × 10 −27 S m 2 in the silicon slow-light PhC-wg, with σ and k c deduced from the empirical expression in Lin et al. [44] The generation of the TPA-induced free carriers obeys the following rate equation where N c ( z,t ) is the free-carrier density and τ c ~0.5 ns is the carrier lifetime [45] . Bright solitons are the analytic solutions to Equation 1 considering only the SPM ( γ ) and anomalous GVD ( β 2 ) terms. In this case, soliton propagation is characterized by two length scales: the dispersion length L D =T 0 2 /| β 2 |, where T 0 =T FWHM /Γ , T FWHM is the full-width half-maximum, Γ =1.665 for Gaussian pulses, with the nonlinear length L NL =1/P 0 γ eff . The soliton number defines the conditions for soliton propagation including slow-light nonlinearity enhancement, S 2 (refs 25 , 26 ). In the canonical case, in which only SPM and GVD are considered, the pulse propagates without dispersing as a fundamental soliton when N =1, while the solutions with N >1 correspond to higher-order solitons. In this latter case, the pulse experiences recurrent periodic evolution by first compressing, then splitting into two distinct peaks, which later re-collide, before finally resuming the initial shape after a soliton period z 0 =(π/2) L D [41] , [42] . The soliton number determines both the maximum achievable compression factor χ c = T in / T out and the point at which it occurs within the soliton period z / z 0 . Efficient soliton compression requires large N values, as this results in superior compression χ c and shorter-length scale z / z 0 (ref. 15 ). The simple canonical description of Equation 3 does not consider TPA, free carriers, linear loss or higher-order dispersion and is therefore an incomplete description of soliton evolution in silicon. Nonetheless, we can use this formalism, along with our knowledge of these ancillary nonlinear processes, to intuitively reason why solitons are difficult to observe in silicon. Achieving a desirable soliton output relies on the precise control of three key parameters: P 0 S 2 , β 2 and T 0 . The nonlinear parameter γ is a constant determined by the material and geometry. The most striking difference in silicon compared with the canonical dynamics is that the P 0 S 2 product saturates due to TPA loss [46] . This term essentially behaves as a constant for large values of P 0 or S , thereby eliminating a key control knob governing the soliton evolution. We are left with only two free parameters to modulate the soliton, T 0 and β 2 , with N 2 proportional to T 0 2 /| β 2 |—that is, the dispersion length L D . As we desire ultracompact chip scale operation, this implies a large value of anomalous dispersion, for which photonic crystals are ideal. Examining Equation 3 further, we notice that a large value of β 2 results in a decrease in N, which is counter to the goal of large N required for efficient compression. Consequently, one must employ long pulses (larger T 0 ) to increase N. The final bound on the system is to make sure that T 0 is not too large, or the soliton period z 0 will require an impractically long device dominated by linear loss. In summary, TPA imposes a unique set of additional restrictions on P 0 S 2 , β 2 and T 0 for soliton compression in silicon. Perhaps even more important than the TPA-loss mechanism is the role of free carriers. The last term of Equation 1 reveals that free carriers interact with the optical pulse by both modulating its phase by FCD (which acts counter to the Kerr effect), as well as reducing intensity by FCA. As dictated by Equation 2, the generation of free carriers in time follows the evolution of the pulse intensity squared—that is, the free-carrier concentration will be negligible at the leading edge of the pulse and be significant at the trailing edge. Therefore, FCA causes nonlinear absorption of the trailing edge of the pulse (red components in anomalous dispersion media), generating pulse asymmetry [46] . Moreover, since the parameter k c,eff in Equation 1 takes negative values, FCD shifts the spectrum towards the blue [47] and, as the dispersion is anomalous, this blue-shifted part of the pulse travels faster, causing pulse acceleration. As a result of its interaction with free carriers, the symmetry of the optical pulse is irreversibly broken and the recurrent soliton evolution cannot occur. Time-resolved measurements of silicon soliton compression In order to demonstrate soliton compression in silicon, we inject 3.7-ps pulses into a 396-μm-long dispersion-engineered silicon PhC-wg, as shown in Fig. 2a (see Methods). 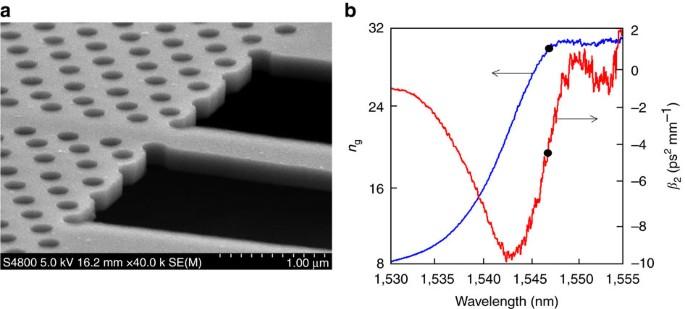Figure 2: Characterization of the dispersion engineered slow-light silicon photonic crystal waveguide. (a) Scanning electron micrograph; (b) group index (blue) and group velocity dispersion parameter (red) measured with an interferometric technique. The dot indicates the operating point of the experiment. Figure 2b shows the dispersion of the PhC-wg measured using an interferometric technique [48] . For the pulse central wavelength of this experiment λ 0 =1,547 nm, the group index n g is 28.5 with β 2 =−4.7 ps 2 mm −1 and β 3 =2.4 ps 3 mm −1 . The dispersion engineering in the sample is absolutely critical to these results as it moves the large dispersion regime away from the bandedge, where the backscattering losses are known to scale with S 2 (ref. 49 ), in contrast to the loss scaling with only S here [50] . Compared to previous results using un-engineered PhC-wgs [51] , created by simply removing a row of holes from the PhC lattice, the sample used in this work avoids the excessive impact of linear loss on the nonlinear induced phase shift. We also note that the mode is guided by the photonic bandgap effect in present regime, which allows for the large variation in β 2 shown in Fig. 2b while keeping the mode area approximately constant [52] . Figure 2: Characterization of the dispersion engineered slow-light silicon photonic crystal waveguide. ( a ) Scanning electron micrograph; ( b ) group index (blue) and group velocity dispersion parameter (red) measured with an interferometric technique. The dot indicates the operating point of the experiment. Full size image For the time-resolved ultra-short pulse characterization we have constructed a phase-sensitive FREG [38] apparatus (see Methods). FREG allows for simultaneous pulse intensity and phase retrieval in both temporal and spectral domains with greatly increased sensitivity, up to 10 −17 J, compared with nonlinear all-optical gating techniques such as frequency-resolved optical gating [53] . In our cross-correlation configuration, we also measure the pulse time of flight. 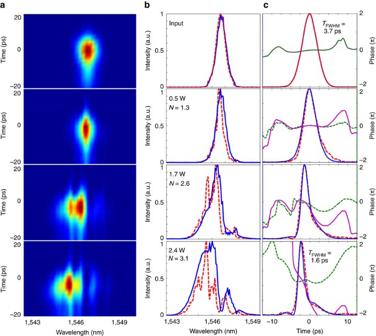Figure 3: Time-resolved measurements of soliton compression. (a) Experimental FREG spectrograms. (b) Measured (dashed red) and modelled (blue) intensity in the spectral domain; (c) measured intensity (dashed red) and phase (dashed green) along with the NLSE-modelled intensity (blue) and phase (magenta) in the time domain following numerical deconvolution. Figure 3a shows the FREG spectrograms (see also Supplementary Movie 1 ) for the input pulse and for the output pulse at three different coupled power levels, along with the associated soliton number, N . The spectrograms clearly reveal the pulse spectrally blue-shifting with increasing power due to larger free-carrier concentrations. The spectrogram cross-correlations are broader in time than the optical pulses due to the ~12-ps electronic gate pulse. Figure 3b,c show the experimentally retrieved pulse intensities in the spectral and time domains, respectively, indicated as the dashed red lines. We confirm these measurements with NLSE modelling (blue line), demonstrating excellent agreement. The retrieved spectral shapes in Fig. 3b illustrate the asymmetry caused by the effect of FCA on the red part of the pulse and by the blue components introduced by FCD [45] . Figure 3: Time-resolved measurements of soliton compression. ( a ) Experimental FREG spectrograms. ( b ) Measured (dashed red) and modelled (blue) intensity in the spectral domain; ( c ) measured intensity (dashed red) and phase (dashed green) along with the NLSE-modelled intensity (blue) and phase (magenta) in the time domain following numerical deconvolution. Full size image In the time domain ( Fig. 3c ) the effect of the free carriers over the trailing edge of the pulse noticeably results in the pulse developing a steep leading edge and getting accelerated in time. More importantly, we observe compression of 3.7-ps pulses to a minimum duration of 1.6 ps (compression factor χ c =2.3) at 2.4 W (~9 pJ), which represents the first experimental demonstration of picosecond pulse soliton compression in silicon. The phase of the 0.5 W case in Fig. 3c is mostly flat, indicating the characteristic balance of SPM and GVD for the fundamental soliton. This case, corresponding to N ~1.3, could be described as a path-averaged fundamental soliton, in which the input peak power needed to get a fundamental soliton ( N =1) is increased by averaging the pulse-peak power over the waveguide [54] . By doing so, we are accounting for the linear and nonlinear loss that the pulse will undergo when propagating over the waveguide length. For this particular case, the peak power averaged over the waveguide is P 0,avg =(1/ L )∫ P 0 ( z )d z =0.35 W. This averaged value gives rise to a path-averaged soliton number of N ~1.1, roughly a fundamental soliton. Figure 3c also shows that the pulse phase is significantly affected by free-carrier dynamics at larger input powers, with strong modulation at positive delay (pulse tail) due to the time-delayed response of the free carriers. We suspect that the discrepancy in the highest power case is due to the formation of a dispersive wave as revealed by the spectrogram [55] . Strong coupling of free carriers and solitons in silicon To gain a deeper understanding of the physics of the measured spectrograms, in Fig. 4 we overlap the spectral blue shift, temporal acceleration and pulse width retrieved from the experimental measurements (blue dots) with the NLSE modelling results (solid black line). The results of the NLSE modelling are in very good agreement with the experimental data for both blue shift ( Fig. 4a ) and acceleration ( Fig. 4b ) as a function of peak power coupled into the PhC-wg. Recall that femtosecond pulses in channel waveguides are too short in temporal duration to experience the free-carrier effects and consequently exhibit negligible acceleration [36] . The black dashed line in Fig. 4a,b indicates simulations in equivalent 3PA media. The acceleration is less noticeable in this simulated case due to an order of magnitude lower free-carrier concentration. Soliton acceleration in silicon clearly requires a careful balance of large carrier concentration characteristic of TPA media (versus 3PA media), anomalous dispersion, as well as pulses of sufficient time duration (picoseconds versus femtoseconds) to experience the FCD in a medium with anomalous dispersion. 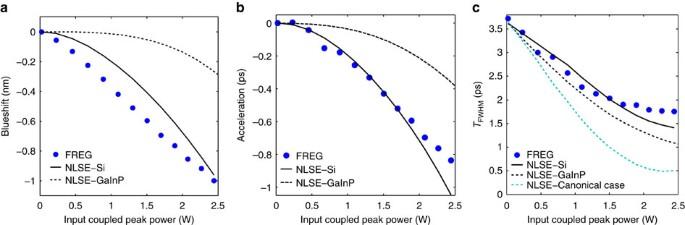Figure 4: Dynamics of the picosecond solitons in silicon. (a) Measured (blue dots) and simulated (black line) blue shift as a function of coupled peak power in silicon. Simulated pulse blue shift in an equivalent 3PA medium with reduced free carriers exhibit smaller soliton-free carrier coupling (dashed black). (b) Measured (blue dots) and simulated (black line) acceleration as a function of coupled peak power in silicon. The pulses in a simulated 3PA medium accelerate much less than silicon (dashed black). (c) Temporal pulse width as a function of the peak power coupled into the photonic crystal waveguide for the measured pulses (blue dots), full-model simulated pulse (black solid line), the 3PA case (black dashed line) and the canonical model of GVD and SPM (dashed turquoise line). Figure 4: Dynamics of the picosecond solitons in silicon. ( a ) Measured (blue dots) and simulated (black line) blue shift as a function of coupled peak power in silicon. Simulated pulse blue shift in an equivalent 3PA medium with reduced free carriers exhibit smaller soliton-free carrier coupling (dashed black). ( b ) Measured (blue dots) and simulated (black line) acceleration as a function of coupled peak power in silicon. The pulses in a simulated 3PA medium accelerate much less than silicon (dashed black). ( c ) Temporal pulse width as a function of the peak power coupled into the photonic crystal waveguide for the measured pulses (blue dots), full-model simulated pulse (black solid line), the 3PA case (black dashed line) and the canonical model of GVD and SPM (dashed turquoise line). Full size image Figure 4c shows the pulse temporal duration retrieved from the FREG measurements as a function of input power (blue dots). The plot indicates stronger pulse compression with increasing power and a tendency to saturate at large powers, in agreement with our NLSE model with all effects taken into account (solid black line)—linear loss, TPA, FCA and FCD. We further simulate the canonical case of SPM and GVD in our model (turquoise dashed line). Comparing this case to the experimental data, it is clear that the presence of TPA and free carriers in our system has reduced the maximum compression factor by a factor of ~3. The simulations in equivalent 3PA media (black dashed line) show compression factors closer to the canonical case due to lower nonlinear loss and weaker interaction of the optical soliton with the free carriers. 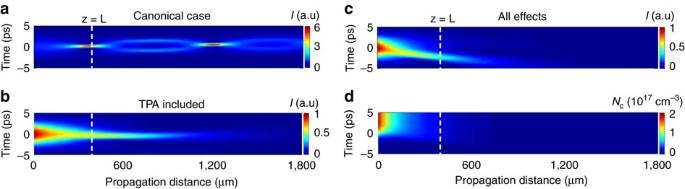Figure 5: Comparison of the canonical soliton with the soliton perturbed by TPA and free carriers. NLSE-modelled normalized temporal intensity as a function of the propagation distance for the higher-power case (2.4 W), (a) considering only the effect of SPM and GVD, (b) considering also higher-order dispersion and TPA, and (c) considering also the absorptive and dispersive effects of free carriers. (d) Free-carrier density as a function of the propagation distance for case (c). Figure 5 illustrates the modelled soliton evolution along our soliton period z 0 ≈1.8 mm for several cases: canonical soliton dynamics ( Fig. 5a ) and the more complex dynamics that arise when TPA ( Fig. 5b ) and its accompanying free carriers ( Fig. 5c,d ) come into play. Figure 5a shows NLSE modelling of higher-order canonical soliton ( N =3.1) periodic evolution along z 0 . The slight asymmetry barely perceivable in Fig. 5a is due to the tiny residual chirp of the input pulse. When TPA is present, as indicated in Fig. 5b , the pulse compression occurs later along the propagation length due to the nonlinear loss mechanism. As a consequence of the power saturation caused by TPA loss, the expected intensity increase associated with pulse compression does not take place anymore. The acceleration is clearly linked to the TPA-induced free carriers as indicated by the contour plots in Fig. 5c,d . Note that the free-carrier density, shown in Fig. 5d , is only significant over the trailing part of the pulse and along the propagation distance where the pulse is intense enough to trigger TPA. Figure 5: Comparison of the canonical soliton with the soliton perturbed by TPA and free carriers. NLSE-modelled normalized temporal intensity as a function of the propagation distance for the higher-power case (2.4 W), ( a ) considering only the effect of SPM and GVD, ( b ) considering also higher-order dispersion and TPA, and ( c ) considering also the absorptive and dispersive effects of free carriers. ( d ) Free-carrier density as a function of the propagation distance for case ( c ). Full size image Here using a slow-light PhC-wg, we have reported the experimental demonstration of compression of 3.7-ps pulses to a minimum duration of 1.6 ps at 9 pJ energy in silicon. The physics governing this result have been thoroughly investigated, with an emphasis on the role of TPA and TPA-induced free carriers. The strong interaction of the on-chip optical solitons and free carriers has been elucidated through an ultra-sensitive phase-resolved FREG technique and confirmed by excellent agreement with NLSE modelling. These observations are due to the careful selection of a huge anomalous dispersion in the dispersion-engineered photonic crystal waveguide, allowing for picosecond soliton evolution in the compact device; a slow-light enhanced Kerr effect, enabling strong nonlinearities at peak powers of only a few watts; and the appropriate selection of the pulse width required to observe compression in the TPA-restricted material. These results further our understanding of nonlinear wave propagation in silicon waveguides, opening the possibility of soliton functionalities for metrology, ultrafast pulses and chip-scale communication systems in a monolithic CMOS platform. Free-carrier schematics The free-carrier schematics of Fig. 1c are generated via nonlinear Schrödinger numerical modelling shown in the main text with suppressed dispersion ( β 2 = β 3 =0). Equal pulse energies (different peak power) were assumed for the pulse inputs. The input pulses are 3.7 ps ( P avg =1,200 μW, P 0 =2.4 W, N =3.1), as in our experiments, and 100 fs ( P avg =1,200 μW, P 0 =40 W, N =0.33), with all other parameters kept constant. The point is to illustrate the difference in chirp between the two regimes, namely that significantly more blue components are generated by picosecond pulses. Device and linear characterization The present experiment was performed using a silicon photonic crystal air-suspended structure with a hexagonal lattice (p6m symmetry group) constant a of 404 nm, a hole radius r of 116 nm and a thickness t of 220 nm, yielding an effective mode area A eff =0.47 μm 2 . A 396-μm-long dispersion-engineered PhC-wg is created by removing a row of holes and shifting the two innermost adjacent rows 50 nm away from the line defect. The air-clad devices were fabricated with a combination of electron beam lithography, reactive ion and chemical wet etching. The measured linear propagation loss in this slow light region is ~70 dB cm −1 , with a total linear insertion loss of ~13 dB (5 dB per facet). Light was coupled in with tapered lensed fibres to SU8 polymer waveguides with inverse tapers. The linear loss in the nanowires that couple light into and out of the PhC-wg is negligible. Nonlinear absorption in the coupling nanowire ( A eff ~0.2 μm 2 ) was taken into account in the NLSE model. Phase-resolved characterization method For the nonlinear experiment, we used a mode-locked-laser (Alnair) fed into a pulse shaper (Finisar) generating near transform-limited 3.7-ps pulses at 1,547 nm at 30-MHz repetition rate. These pulses are then input into the FREG [38] apparatus. The pulses are split into two branches by a fibre coupler, with the majority of the energy coupled into the PhC-wg. The remaining fraction is sent to a reference branch with a variable delay, before being detected by a fast photodiode and transferred to the electronic domain. This electronic signal drives a Mach–Zender modulator that gates the optical pulse output from the PhC-wg. Using an optical spectrum analyser, we measure the spectra as a function of delay to generate a series of optical spectrograms. We deconvolve the spectrograms with a numerical algorithm (256 × 256 grid-retrieval errors G <0.005), to retrieve the pulse intensity and the phase in both the temporal and spectral domain [56] . How to cite this article: Blanco-Redondo, A. et al. Observation of soliton compression in silicon photonic crystals. Nat. Commun. 5:3160 doi: 10.1038/ncomms4160 (2014).